A scanning transmon qubit for strong coupling circuit quantum electrodynamics Like a quantum computer designed for a particular class of problems, a quantum simulator enables quantitative modelling of quantum systems that is computationally intractable with a classical computer. Superconducting circuits have recently been investigated as an alternative system in which microwave photons confined to a lattice of coupled resonators act as the particles under study, with qubits coupled to the resonators producing effective photon–photon interactions. Such a system promises insight into the non-equilibrium physics of interacting bosons, but new tools are needed to understand this complex behaviour. Here we demonstrate the operation of a scanning transmon qubit and propose its use as a local probe of photon number within a superconducting resonator lattice. We map the coupling strength of the qubit to a resonator on a separate chip and show that the system reaches the strong coupling regime over a wide scanning area. Over the past decade, the study of quantum physics using superconducting circuits has seen rapid advances in sample design and measurement techniques [1] , [2] , [3] . A great strength of superconducting qubits compared with other promising controlled quantum systems is that they are fabricated using standard lithography procedures, which allow fine tuning of qubit properties and make scaling up the fabrication to devices with many qubits straightforward. Circuit quantum electrodynamics (CQED) is an active branch of quantum physics research in which one or more qubits are strongly coupled to a superconducting coplanar waveguide resonator (CPWR), which is used to control and read out the state of the qubits [4] , [5] . A prerequisite for most interesting CQED applications is that the system reach the strong coupling regime in which the rate at which the qubit and the resonator exchange an excitation exceeds the excitation decay rate [5] , [6] . Although the CQED architecture has primarily been studied as a quantum computing platform, recent theoretical work has focused on using a CQED lattice, a network of coupled resonators each coupled to its own qubit, as a non-equilibrium quantum simulator [7] . One particularly interesting prediction for CQED lattice systems is a cross-over from a superfluid-like state to an insulating state as, for example, the coupling between the qubits and their resonators is increased [8] , [9] , [10] , which is similar to the superfluid-Mott insulator quantum-phase transition that has been observed in ultracold atom systems [11] , [12] . More exotic phenomena including analogues of the fractional [13] and anomalous [14] quantum Hall effects and of Majorana physics [15] have also been considered. However, while preliminary steps have been taken to build such a CQED lattice system [16] , both establishing and probing its expected many-body states remain major experimental challenges. The simplest method of probing a microwave circuit is to measure the transmission between two of its ports. However, in the case of a CQED lattice such a measurement gives only limited insight into the detailed behaviour of photons in the interior. Additional information could be obtained by measuring transmission while locally perturbing the interior of the sample, as has been done to image the coherent flow of electrons in two-dimensional electron gas systems [17] , [18] . This local perturbation requires a new scanning tool, such as the scanning qubit demonstrated here. Besides just perturbing the lattice, a scanning qubit can be used to measure the photon number of individual lattice sites, following a protocol used to measure photons in non-scannable cavities [19] . One benefit of a scanning qubit in this case is its ability to measure the photon number of interior lattice sites. Measurements of outer resonators, those most easily accessed by a measurement circuit fabricated on the same chip as the lattice, would be difficult to interpret due to edge effects. Although our primary focus is on using the scanning qubit in the context of CQED lattice-based quantum simulation, we note that scanning qubits have been studied previously for other applications. Scanning nitrogen-vacancy (NV) centre qubits in diamond have been demonstrated to be sensitive local probes of magnetic field [20] , [21] . An important feature of NV centers is their atomic size scale, which allows them to be incorporated into imaging systems capable of nanometer-scale resolution. In order to be compatible with typical superconducting quantum circuits, the transmon qubit described here has micrometre scale features and thus provides much less spatial resolution. An NV centre has also been coupled to a scanning photonic crystal cavity [22] . Although this experiment did not reach the strong coupling regime, the scanning cavity enhanced spontaneous emission from the NV centre and allowed its position to be determined with greater spatial resolution. In this work, we describe a scanning superconducting qubit and demonstrate its coupling to a superconducting CPWR on a separate chip. The strength of the coupling between the resonator and the qubit is mapped out over a 0.25 × 2.4 mm 2 area around the resonator. The qubit and resonator decay rates are found to be reasonably low, allowing the system to enter the strong coupling regime for most of this area. We propose this qubit’s use as a scannable probe of a CQED lattice system and more broadly as a qubit with in situ tunable coupling to a resonator. Experimental setup The scanning qubit described here ( Fig. 1 ) is a transmon design consisting of two aluminium islands connected by a thin aluminium wire interrupted by an aluminium oxide tunnel barrier [23] . The tunnel barrier provides a large nonlinear inductance which, together with the capacitance between the two islands, makes the transmon behave as a nonlinear LC oscillator, whose lowest two energy states can be used as a qubit. The transmon design is well suited for scanning because it couples to CPWRs capacitively and requires no physical connections. The qubit chip was mounted face down to a cryogenic three-axis positioning stage, and positioned over a separate chip containing a niobium CPWR with a half-wave resonance at 7.6 GHz. In order to avoid direct contact between the resonator and the qubit, pads of photoresist 7 μm thick were deposited on the corners of the qubit chip. The sample holder was mounted to a dilution refrigerator that operated at temperatures 35 mK. 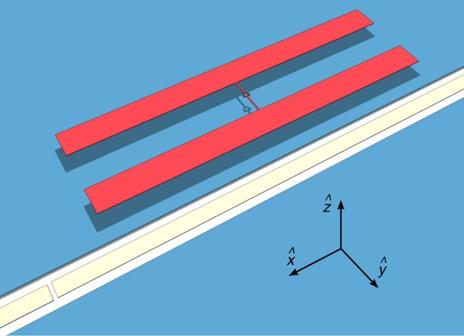Figure 1: Scanning transmon qubit. The qubit (red) is composed of two 40 × 500 μm2aluminium islands separated by a 60 μm gap and connected by a thin wire containing a Josephson tunnel barrier. In the qubit discussed here, the tunnel barrier is formed by two aluminium oxide barriers in the two arms of a loop in the middle of the wire. The qubit is pictured 11 μm above a portion of a CPWR. The resonator’s centre pin (yellow) is 21 μm wide and is separated from the surrounding ground plane (blue) by 12 μm gaps. The ends of the resonator are formed by gaps in the centre pin like the one shown in the figure. The resonator has a length of 7,872 μm, which corresponds to a half-wave resonance of 7.6 GHz in the absence of the qubit. The resonator centre pin has no curves in over half its length, so that the qubit remains aligned as it scans over this part of the resonator. To make them more visible, the qubit and resonator have been thickened, but all other dimensions are to scale with the samples discussed here. Figure 1: Scanning transmon qubit. The qubit (red) is composed of two 40 × 500 μm 2 aluminium islands separated by a 60 μm gap and connected by a thin wire containing a Josephson tunnel barrier. In the qubit discussed here, the tunnel barrier is formed by two aluminium oxide barriers in the two arms of a loop in the middle of the wire. The qubit is pictured 11 μm above a portion of a CPWR. The resonator’s centre pin (yellow) is 21 μm wide and is separated from the surrounding ground plane (blue) by 12 μm gaps. The ends of the resonator are formed by gaps in the centre pin like the one shown in the figure. The resonator has a length of 7,872 μm, which corresponds to a half-wave resonance of 7.6 GHz in the absence of the qubit. The resonator centre pin has no curves in over half its length, so that the qubit remains aligned as it scans over this part of the resonator. To make them more visible, the qubit and resonator have been thickened, but all other dimensions are to scale with the samples discussed here. Full size image Qubit-resonator coupling strength measurement procedure The main result presented here is the measurement of the strength g of the coupling between the resonator and the qubit as a function of qubit position. Following Koch et al . [23] , the Hamiltonian Ĥ describing the coupled resonator–qubit system can be approximated by the Jaynes–Cummings Hamiltonian with ν r and ν q the resonator and qubit frequencies, respectively. In this expression, â , â † are the creation and annihilation operators associated with photons in the resonator, and , and are the Pauli spin matrices associated with the qubit when treated as a two-level system. On resonance ( ν q = ν r ), the first two excited states of the system are with corresponding energies hν r ± hg above that of the ground state |0↓ , where | nq is the state with n photons in the resonator and the qubit in state q with ↓(↑), representing the qubit ground (excited) state. When driven with a microwave excitation, transitions to each of these excited states are allowed, resulting in two peaks in the low power transmission spectrum. The coupling between the qubit and the resonator is determined by observing the frequency splitting 2 g of these peaks, which is known as the vacuum Rabi splitting. The frequency ν r of the resonator increases when the qubit chip is brought into close proximity with it. In order to ensure that resonance was possible at every qubit position, the qubit was fabricated with a pair of tunnel barriers integrated into a loop in place of a single-tunnel barrier. By varying the flux through this loop with a magnet coil incorporated into the positioner, the qubit frequency ν q could be varied from a maximum value of 12.1 GHz to close to zero [23] . Although here the flux loop’s only purpose is to make the qubit energy tunable, such a loop can also be operated as a sensitive local magnetometer in a scanning SQUID microscope [24] . Although it is necessary to bring the resonator–qubit system into resonance in order to infer the coupling strength from the vacuum Rabi splitting, many CQED experiments, including the photon number measurement described in Johnson et al . [19] , are performed with the qubit frequency detuned several hundred megahertz from the resonator. In this dispersive regime precise tuning of the qubit frequency is not required, and the qubit can be fabricated with a single-tunnel barrier and measured without an external magnetic field. 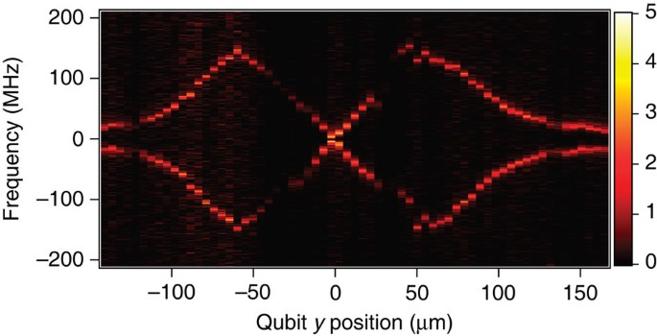Figure 2: Resonant transmission spectra. Transmission spectra taken with the qubit in resonance with the resonator are shown for a series of qubit positions. The vertical axis represents the difference between the frequency of the applied microwave drive and the resonator frequency. The shifted peak locations can also be interpreted as values of the coupling strengthg,which is equal to half the peak separation. We take theyorigin to be the point of smallest peak separation, which we interpret as the position where the qubit is centred over the resonator. The colour represents the magnitude of microwave transmission and is plotted in arbitrary units, as the total gain and loss within the measurement chain has not been calibrated. The suppressed transmission at positionsy=±30 and ±125 μm is due to coupling between the resonator and a parasitic resonance in the metal frame of the qubit chip (seeSupplementary Note 2). Position dependence of qubit-resonator coupling Figure 2 shows the transmission spectra of the resonator for a sequence of regularly spaced qubit positions along the y axis perpendicular to the long dimension of the resonator. At each position, the current through the magnet coil was adjusted to bring the qubit into resonance ( Supplementary Note 1 ), at which point the single transmission peak of the resonator was transformed into two peaks of equal height, clearly demonstrating strong coupling between the scanning qubit and the resonator. The position scan shows two regions of large peak separation that are symmetric about a position with nearly no peak separation, which we set as the origin. In coupling to the resonator the transmon behaves as a dipole antenna. Because the two islands of the qubit are identical, by symmetry no coupling is expected when the qubit is centred above the resonator at y =0. The points of maximum peak separation occur at y ≈±50 μm, where one of the two islands is centred over the resonator. At these points, the observed coupling strength g ≈140 MHz was well into the strong coupling regime where the qubit relaxation time T 1 =3.2 s was determined by time-domain measurements (see Methods) and the photon escape rate κ =10 MHz was set by the resonator’s output coupling capacitor, which was chosen to be large in order to increase the rate of data acquisition. The photon escape rate κ , proportional to the linewidth of the transmission peak, was relatively constant as a function of position, except for positions where a parasitic mode coupled to the resonator and broadened the linewidth to as much as 35 MHz ( Supplementary Note 2 ). Figure 2: Resonant transmission spectra. Transmission spectra taken with the qubit in resonance with the resonator are shown for a series of qubit positions. The vertical axis represents the difference between the frequency of the applied microwave drive and the resonator frequency. The shifted peak locations can also be interpreted as values of the coupling strength g, which is equal to half the peak separation. We take the y origin to be the point of smallest peak separation, which we interpret as the position where the qubit is centred over the resonator. The colour represents the magnitude of microwave transmission and is plotted in arbitrary units, as the total gain and loss within the measurement chain has not been calibrated. The suppressed transmission at positions y =±30 and ±125 μm is due to coupling between the resonator and a parasitic resonance in the metal frame of the qubit chip (see Supplementary Note 2 ). Full size image Scans of resonant transmission versus y position, such as Fig. 2 , were repeated at five positions along the length of the resonator (the direction) with a spacing of 600 μm. The coupling strengths g extracted from fits to the transmission spectrum at each qubit position ( Supplementary Methods ) are plotted in Fig. 3 . The coupling strength increases as the qubit moves from the voltage node at the centre of the resonator to the antinode at its end but exhibits the same shape for its y dependence at each x position. For technical reasons related to the operation of the positioning stage, measurements of the coupling strength at different z positions were not performed ( Supplementary Note 3 ). 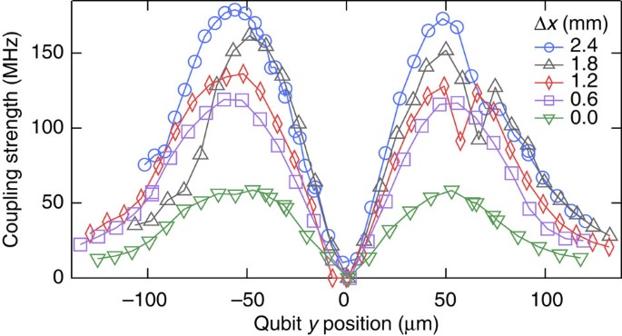Figure 3: Coupling strengthgversus qubit position. Traces ofgversus qubityposition are shown for five qubitxpositions spaced 600 μm apart from each other. The traces correspond to scans, such as the one shown inFig. 2. Each value ofgwas determined by fitting several transmission spectra taken at values of magnetic flux for which the qubit frequency was close to that of the resonator. The sign of Δxis such that with increasing Δxthe qubit moves from the electric field node at the centre of the resonator towards the electric field antinode at its end. The individual coupling strength values betweeny=55 and 80 μm that deviate from the smooth trends ofgversusyfor Δx≥1.2 mm correspond to positions where the resonator coupled to a parasitic mode in the metal frame of the qubit chip (seeSupplementary Note 2). Figure 3: Coupling strength g versus qubit position. Traces of g versus qubit y position are shown for five qubit x positions spaced 600 μm apart from each other. The traces correspond to scans, such as the one shown in Fig. 2 . Each value of g was determined by fitting several transmission spectra taken at values of magnetic flux for which the qubit frequency was close to that of the resonator. The sign of Δ x is such that with increasing Δ x the qubit moves from the electric field node at the centre of the resonator towards the electric field antinode at its end. The individual coupling strength values between y =55 and 80 μm that deviate from the smooth trends of g versus y for Δ x ≥1.2 mm correspond to positions where the resonator coupled to a parasitic mode in the metal frame of the qubit chip (see Supplementary Note 2 ). Full size image Comparison with simulation We now consider the data in Fig. 3 more quantitatively. The coupling strength g is proportional to the electric field at the position of the qubit produced by a single photon in the resonator. 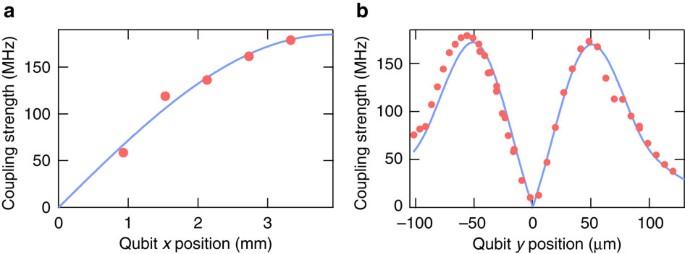Figure 4: Quantitative analysis of measured coupling strength. (a) The maximum coupling strengthgof each trace inFig. 3is plotted versusxposition along with a fit to the expected sinusoidal dependence. Thexorigin represents the midpoint of the resonator. The offset of the data points from the resonator midpoint was determined by the fit (see Methods). The other fit parameter, the maximum coupling strength the end of the resonator, was found to be 185 MHz. (b) The largest trace ofgversusyinFig. 3is replotted along with a fit to the form expected from finite element modelling of the qubit-resonator system’s capacitance matrix (see Methods). The fitting function uses the resonator frequencyνr, the system geometry, and the qubitxposition determined in panelaas fixed inputs and treats the qubit heightz, found to be 11 μm, as its only free parameter. Figure 4a shows the maximum value of g for each x position along with a fit to the expected sinusoidal dependence of the electric field strength. The fit provides an absolute reference for the relative x positions quoted in Fig. 3 . With the x position known, we can compare the measurement data with the g ( x , y , z ) obtained from finite element simulations (see Methods). Figure 4: Quantitative analysis of measured coupling strength. ( a ) The maximum coupling strength g of each trace in Fig. 3 is plotted versus x position along with a fit to the expected sinusoidal dependence. The x origin represents the midpoint of the resonator. The offset of the data points from the resonator midpoint was determined by the fit (see Methods). The other fit parameter, the maximum coupling strength the end of the resonator, was found to be 185 MHz. ( b ) The largest trace of g versus y in Fig. 3 is replotted along with a fit to the form expected from finite element modelling of the qubit-resonator system’s capacitance matrix (see Methods). The fitting function uses the resonator frequency ν r , the system geometry, and the qubit x position determined in panel a as fixed inputs and treats the qubit height z , found to be 11 μm, as its only free parameter. Full size image Figure 4b shows the values of g observed for x =3,330 μm from the resonator midpoint along with the simulation results, which show good agreement. The simulation height z =11 μm is somewhat larger than the 7 μm thickness of the photoresist pads on the corners of the qubit chip but corresponds to a misalignment between the qubit and resonator chips of ~0.1° over 2 mm distance from the edge of the qubit chip to the qubit’s location at the chip centre. Such a misalignment could cause one island of the qubit to be 0.4 μm higher than the other. This height difference would cause the coupling strength to be as much as 1% stronger for a given y compared with its value at − y . Asymmetry in the qubit chip design (see Methods) is responsible for an additional 1% asymmetry. Together, these two sources of asymmetry come close to accounting for the observed 3% asymmetry in the measured values of g plotted in Fig. 4b . We attribute the apparent disagreement in y between the observed g and the simulation to drift in the reading of the positioning stage (see Methods). We have observed strong coupling between a scanning transmon qubit and a CPWR. Because strong coupling can be reached, anything possible with stationary qubits now becomes possible with a moveable probe opening the door for a wide array of applications in the field of CQED. Such a scanning qubit makes possible quantum measurements of superconducting circuits with spatial resolution. In addition to the scanning measurements of a lattice CQED system discussed earlier, we note that the system studied here demonstrates in situ tuning of the coupling strength g, which is often a desirable capability experimentally. Although the scanning qubit’s coupling cannot be tuned on the timescale of the coherence time like some previously demonstrated circuit designs [25] , [26] , it does not require flux or current biasing of the system. For example, for the lattice CQED system mentioned above, a lattice of resonators on one chip could be coupled to a lattice of qubits on a second chip, thus allowing the coupling between each resonator–qubit pair to be tuned together as one chip is scanned over the other. An array of qubits could also be used to measure the statistics of qubit coherence by scanning the qubits one by one across a single-measurement resonator. Sample fabrication The qubit was fabricated using electron beam lithography and double-angle shadow evaporation with controlled oxidation of 30 and 100 nm layers of aluminium onto a 4 × 4 mm 2 sapphire chip. The 0.5 × 1.0 mm 2 crashpads on the corners of the chip were made with photolithography of SU-8 2005 photoresist. The resonator was defined by photolithography and acid etch (H 2 O, HF and HNO 3 in a 7.5:4:1 ratio) of a 200 nm film of niobium on a 14 × 14 mm 2 sapphire chip. Sample mounting and wiring The qubit chip was glued with methyl methacrylate to the tip of a highly conductive copper rod mounted to the cryogenic positioning stage (Attocube ANPx340/RES, ANPz101/RES). The resonator chip was mounted to a copper-patterned circuit board with silver paste and aluminium wire bonds, which connected the input and output transmission lines to coaxial lines. Wire bonds were only placed around the edge of the chip outside the footprint of the qubit chip. The wiring scheme of the coaxial lines was the same as that described in DiCarlo et al . [27] . Qubit positioning All values of qubit position were determined by potentiometric measurements of resistive position encoders integrated into the positioning stage. Individual position readings had an uncertainty of 0.4 μm, and overall the position readings drifted by 1.8 μm per 100 μm. A typical movement of the positioning stage of 10 μm heated the refrigerator from its base temperature of 15 mK to over 85 mK. In order to reduce measurement time, most measurements were taken with the refrigerator in the range between 25 and 35 mK, which took only a couple minutes to reach after moving the stage. Coherence measurements Qubit coherence times ( T 1 =3.2±0.1 μs, μs) were obtained using the techniques described in Schreier et al . [28] For T 1 , the qubit was driven into the excited state by a pulse slightly detuned from the qubit frequency with detuning Δ~10 MHz and then measured with a pulse at the cavity frequency at a delay time τ after the qubit pulse. The excited state probability obtained from many averages for a series of values of τ was fit to a decaying exponential with time constant T 1 . For , the qubit was excited by a pulse with half the height of the pulse that drove the qubit into the excited state and excited again with a second identical pulse after a delay time τ . Then the qubit state was measured. The value of was obtained by fitting the qubit excited state probability to an exponentially decaying sinusoid with frequency Δ and decay constant . The measurements were made during the same cooldown and at the same x position as the data shown in Fig. 2 . For technical reasons, the measurements were made immediately after the refrigerator was warmed up to 20 K and then cooled back down to its base temperature. The coherence measurements were performed at y =−113 μm ( g =31 MHz) in Fig. 2 with the qubit frequency detuned 700 MHz below the resonator. Coupling strength versus x The voltage profiles of the modes of a CPWR with open boundary conditions are sinusoidal along the length of the resonator with antinodes at its ends. The coupling strength is proportional to the resonator voltage with one photon present and so should follow this sinusoid. The maximum coupling strength at each x position shown in Fig. 4a was fit to the sinusoidal form: where l r =7,872 μm is the resonator length and g max and x 0 were the fitting parameters. Here Δ x is the set of displacements in x from the first x position (that is, the values are 0 μm; 600 μm; 1,200 μm and so on). In Figure 4a , the measured coupling strengths and the fit are plotted versus x =Δ x + x 0 . The scan shown in Fig. 2 was taken on a separate cooldown from the scans shown in Fig. 3 . The same resonator and qubit samples were used for both sets of measurements, but the sample stage was disassembled in between the cooldowns. During the cooldown in which data in Fig. 2 was taken, the qubit’s x position was not varied, so the absolute x position of the data is not known. However, using the maximum value of g from Fig. 2 and the curve shown in Fig. 4a to calibrate the x position, one finds the data in Fig. 2 was taken at x =2,116 μm. Coupling strength versus y In order to perform the fit of coupling strength versus y shown in Fig. 4b , the following expression for the coupling strength given in Koch et al . [23] was used: with the characteristic line impedance Z c taken to be 50 Ω and m ( x ) the sinusoidal mode shape factor given in equation (2). In order to describe the voltage division factor β and the transmon matrix element n 01 , we first define C jk to be the capacitance between components j and k and label the components of the system with a and b for the two islands of the transmon, p for the resonator centre pin and g for all other pieces of metal (the two ground planes and the metal frame on the qubit chip). The voltage division factor β gives the fraction of the voltage drop from the resonator centre pin to ground that falls across the two islands of the qubit. It can be written in terms of capacitance coefficients as where C Σ, x = C x p + C x g . We find the matrix element n 01 by numerically diagonalizing the transmon Hamiltonian given in Koch et al . [23] to finds its eigenstates and eigenenergies, and then evaluating , where |0› and |1› are the eigenstates with the two lowest energies, E 0 and E 1 . The charging energy E C = e 2 /2 C Σ was calculated using the total capacitance given by The qubit frequency ν q is given by ( E 1 — E 0 )/ h and is thus a function of E C and E J . In calculating n 01 , ν q ( E C , E J ) was numerically inverted to solve for E J ( E C , ν q ) with ν q set equal to ν r , as measurements of the coupling strength were made with the qubit close to the resonator’s frequency. In order to produce the fit shown in Fig. 4b , the coupling strength g ( x , y , z ) was calculated using the known values of Z c and ν r , the value of x obtained from the fit in Fig. 4a , and the values of the capacitances C jk found by finite element analysis for a grid of y and z values with 1 μm spacing. The measured coupling strength versus y was fit to the g ( y , z ) found by interpolating between the y and z grid points with z as the only free parameter. The finite element simulation was then repeated with the fitted value of z in order to produce the curve shown in Fig. 4b . We note that at the fitted value of z =11.0 μm the charging energy E C =388 MHz is similar to the values used in other CQED experiments and corresponds to a ratio of E J / E C =59, within the transmon regime where the offset charge across the transmon islands (not included in the Hamiltonian given above) may be ignored. The finite element simulation included a layer of metal on the qubit chip that was not symmetric about the qubit and resulted in a asymmetry about y =0 with the value of g at − y being about 1% larger than the value at + y . By the use of alignment marks on the resonator and qubit chips, it was possible to confirm that the misalignment between the two chips in the xy plane was 3°±1°. A misalignment of 3° was used in the finite element calculations for the capacitance coefficients. Using a misalignment of 2° (4°) instead gave a the fitted height z of 11.1 μm (10.7 μm). How to cite this article: Shanks, W. E. et al . A scanning transmon qubit for strong coupling circuit quantum electrodynamics. Nat. Commun. 4:1991 doi: 10.1038/ncomms2991 (2013).